Dirac Cones in two-dimensional conjugated polymer networks Linear electronic band dispersion and the associated Dirac physics has to date been limited to special-case materials, notably graphene and the surfaces of three-dimensional (3D) topological insulators. Here we report that it is possible to create two-dimensional fully conjugated polymer networks with corresponding conical valence and conduction bands and linear energy dispersion at the Fermi level. This is possible for a wide range of polymer types and connectors, resulting in a versatile new family of experimentally realisable materials with unique tuneable electronic properties. We demonstrate their stability on substrates and possibilities for doping and Dirac cone distortion. Notably, the cones can be maintained in 3D-layered crystals. Resembling covalent organic frameworks, these materials represent a potentially exciting new field combining the unique Dirac physics of graphene with the structural flexibility and design opportunities of organic-conjugated polymer chemistry. The electronic structure of pristine graphene has conical bands, so-called ‘Dirac cones’, which touch at the Fermi level at the K and K′ points in the Brillouin zone [1] . As a result, charge carriers in graphene behave as massless relativistic particles described by the Dirac equation, giving rise to a spectacular range of new physics [2] . This electronic structure is a direct result of the underlying hexagonal symmetry of the two symmetrically equivalent sublattices [3] . However, the inherent simplicity of the graphene lattice, with each sublattice represented by just a single carbon atom in the unit cell, limits the possibilities for structural modification. This has led to an ongoing search for new materials with Dirac charge carriers, for example, through lattice reorganization at surfaces of three-dimensional (3D) topological insulators. Other recent propositions include graphyne, graphdiyene and their hydrogenated counterparts [4] , [5] . Nonetheless to date, ‘Dirac materials’ remain a limited set of special cases, and it would be desirable to find a general, flexible alternative. We propose here a broad family of experimentally realizable two-dimensional (2D) networks of conjugated polymers, which demonstrate graphene-like electronic structure. Their functionality and properties, such as the carrier Fermi velocity, can be customized through appropriate monomer design. Owing to their accessibility to chemical design, these materials have the potential to open up a range of applications not available to graphene. 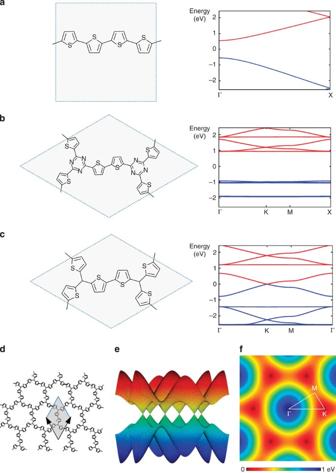Figure 1: Electronic structure change from 1D- to 2D-polymer networks. (a) PTh, an infinite 1D polymer chain, gives a finite band gap at gamma due to Peierls distortion along the backbone. (b) A 2D PTh-derived covalent organic framework. Thiophene oligomers are connected in a hexagonal network via 1,3,5-triazine, resulting in a wide-gap semiconductor material. (c–f) Example of the family of new proposed 2D-CPs (2D-conjugated polymers). In this example thiophene oligomers are connected in a hexagonal network via conductive connectors; here, trivalent carbon atoms (2D-C-(Th2)3). The resultant hexagonal network (d) is conductive, exhibiting a graphene-like band structure with Dirac cones at the Fermi level (e,f). The band structure for polyacetylene (PA), PTh and 2D-C(Th2)3are calculated with different levels of theory: LDA shown here and HSE06 inSupplementary Fig. 3. The calculated band gap for PA and PTh agrees with previous theoretical67and experimental6,68lines of work. Bond lengths for structures A, B and C are given inSupplementary Fig. 1for clarity. The colour scale varies from dark red at the Fermi level to dark blue at +1 eV. 2D-conjugated polymers and the Dirac cone Figure 1 shows the electronic band structure of one of the most common one dimensional (1D) conjugated polymers, polythiophene (PTh). Although the symmetric structure is metallic with dispersed states, a Peierls distortion opens a band gap, rendering the polymer semiconducting (2.0 eV experimentally [6] , [7] ). Conjugated polymers have already been successfully connected into 2D networks creating covalent-organic frameworks (COFs) [8] . An example is shown in Fig. 1b using a trivalent 1,3,5-triazine connecting group. 2D COFs can now be synthesized using dynamic covalent chemistry in milligram quantities [9] via polycondensation of organic monomers, with solvothermal [10] , microwave [11] , [12] and ionothermal [13] , [14] synthesis in solution or directly as monolayers on metallic [15] and graphitic [16] , [17] substrates. Solution-based mono- and few-layer sheets can now be produced at micron diameters, highly crystalline [18] and largely defect-free [19] . These materials demonstrate the incredible capability of modern chemistry to create ‘bottom-up’ uniform repeatable 2D networks from custom-designed monomers [20] , [21] , [22] . However, while 2D COFs appear a promising route to create hexagonal organic monolayers, these materials are wide gap semiconductors [23] , [24] . This is because, while the backbones are frequently conjugated, there is a lack of conjugation through the trivalent connectors. Figure 1: Electronic structure change from 1D- to 2D-polymer networks. ( a ) PTh, an infinite 1D polymer chain, gives a finite band gap at gamma due to Peierls distortion along the backbone. ( b ) A 2D PTh-derived covalent organic framework. Thiophene oligomers are connected in a hexagonal network via 1,3,5-triazine, resulting in a wide-gap semiconductor material. ( c – f ) Example of the family of new proposed 2D-CPs (2D-conjugated polymers). In this example thiophene oligomers are connected in a hexagonal network via conductive connectors; here, trivalent carbon atoms (2D-C-(Th 2 ) 3 ). The resultant hexagonal network ( d ) is conductive, exhibiting a graphene-like band structure with Dirac cones at the Fermi level ( e , f ). The band structure for polyacetylene (PA), PTh and 2D-C(Th 2 ) 3 are calculated with different levels of theory: LDA shown here and HSE06 in Supplementary Fig. 3 . The calculated band gap for PA and PTh agrees with previous theoretical [67] and experimental [6] , [68] lines of work. Bond lengths for structures A, B and C are given in Supplementary Fig. 1 for clarity. The colour scale varies from dark red at the Fermi level to dark blue at +1 eV. Full size image In the current study we explore a wide range of 2D conjugated polymer networks via density functional (DFT) calculations, revealing that the electronic behaviour of such 2D networks changes radically when conducting connecting groups are used. An example is shown in Fig. 1c,d , where thiophene dimers are instead connected in a hexagonal array via trivalent carbon atoms (bond lengths in Supplementary Fig. 1 ). The resultant band structure shows a remarkable resemblance to that of graphene ( Fig. 1c–f ), behaving as a zero gap semiconductor with two inequivalent Dirac cones, with associated linear dispersion at the K and K′ points on the boundary of the first Brillouin zone. Plotting the highest occupied molecular orbital (HOMO) and lowest unoccupied molecular orbital (LUMO) at the Fermi level confirms that the states are dispersed across the whole structure, unlike conventional 2D COFs ( Fig. 2 ). 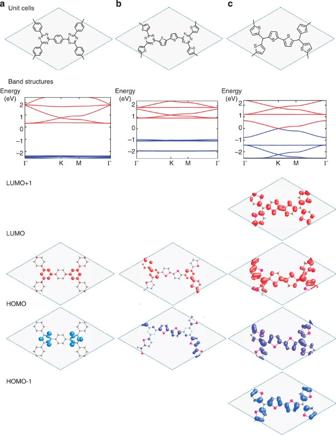Figure 2: Electron distribution in 2D-CPs and COFs. (a) CTF-1, a triazine-based COF (2D-(C3N3)-PP2in our notation), gives a wide-gap semiconductor material, the HOMO (blue-left) and LUMO (red-left) states are localized on the triazine connectors. (b) A 2D polythiophene-derived COF (2D-(C3N3)-PTh2). Thiophene oligomers connected via 1,3,5-triazine, resulting in a wide-gap semiconductor material, the HOMO (blue-centre) and LUMO (red-centre) states are localized on the thiophene oligomers or the triazine connector. (c) Thiophene oligomers connected via a trivalent carbon atom (2D-C-PTh2) exhibiting a graphene-like band structure with Dirac cones at the Fermi level, the HOMO (blue-right) and (red-right) states are delocalized throughout the structure. The HOMO−1 and LUMO+1 states show nodes in the wavefunction on the connectors. All real-space wavefunction plots are for the wavefunction at K in the Brillouin zone. Figure 2: Electron distribution in 2D-CPs and COFs. ( a ) CTF-1, a triazine-based COF (2D-(C 3 N 3 )-PP 2 in our notation), gives a wide-gap semiconductor material, the HOMO (blue-left) and LUMO (red-left) states are localized on the triazine connectors. ( b ) A 2D polythiophene-derived COF (2D-(C 3 N 3 )-PTh 2 ). Thiophene oligomers connected via 1,3,5-triazine, resulting in a wide-gap semiconductor material, the HOMO (blue-centre) and LUMO (red-centre) states are localized on the thiophene oligomers or the triazine connector. ( c ) Thiophene oligomers connected via a trivalent carbon atom (2D-C-PTh 2 ) exhibiting a graphene-like band structure with Dirac cones at the Fermi level, the HOMO (blue-right) and (red-right) states are delocalized throughout the structure. The HOMO−1 and LUMO+1 states show nodes in the wavefunction on the connectors. All real-space wavefunction plots are for the wavefunction at K in the Brillouin zone. Full size image The structure can be understood as a hexagonal array of coupled connectors superposed on a network of conjugated oligomers. The HOMO and LUMO states are originally associated with the radicalar p z orbital on the trivalent connectors. While these states remain primarily localized on the trivalent connectors, they also show character across the conjugated states of the oligomers ( Fig. 2 ). This allows electronic coupling and associated dispersion between the network of trivalent connectors, creating the ‘Dirac cone’ HOMO and LUMO electronic states at the Fermi level. The HOMO-1 and LUMO+1 electronic states come from the conjugated oligomers ( Fig. 2 ). The wavefunctions have nodes at the connectors, rendering them nondispersive and giving rise to flat bands whose separation is controlled by the choice of oligomer (see Table 1 ). Table 1 Electronic band gap of oligomers in 2D-CPs. Full size table This electronic behaviour is remarkably general. The thiophene-based structure shown above is not unique, but instead is simply one example from an entirely new family of 2D-conjugated polymers (2D-CPs), which, unlike COFs, contain conducting connectors. This can be demonstrated with many different conjugated polymers (some examples are given in Fig. 3 ), as well as different conducting connectors. Hereafter, we adopt the notation 2D- a-r 1–3 to describe a hexagonal array of connectors a interlinked with oligomer chains r (nonhexagonal architectures are discussed later). Thus, graphene is the limiting case a =C, r 1–3 =0 (2D-C), and the structure in Fig. 1c is (2D-C-(Th 2 ) 3 ). 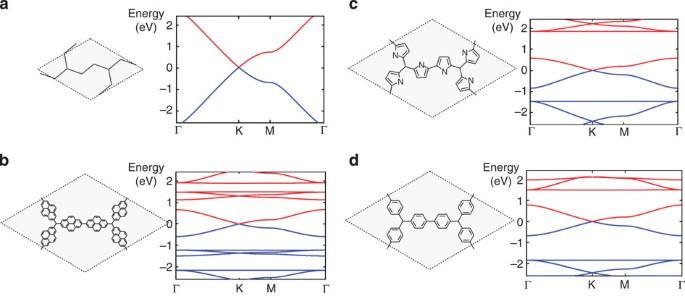Figure 3: Varying the conjugated polymer. Examples of different conjugated polymer backbones in 2D-conjugated polymer hexagonal arrays, using trigonal carbon as the connecting unit, with their corresponding electronic band structures, (a) polyacetylene (PA)-based-C-A3, (b) polypyrene (PPyr)-based 2D-C-Pyr3, (c) polypyrrole (PPy)-based 2D-C-(Py2)3, (d) Poly(p-phenylene) (PPP)-based 2D-C-(PP2)3. The singly occupiedpzstate on each of the two identical carbon atoms in the unit cell act to create linear crossing bands at the Fermi level, creating a Dirac cone as for graphene. Note the oligomers are nonplanar (dihedral angles of 2D-C-A3=12°, 2D-C-Pyr3=30°, 2D-C-(Py2)3=18°, 2D-C-(PP2)3=30°, 2D-C-Th3=21°). Figure 3: Varying the conjugated polymer. Examples of different conjugated polymer backbones in 2D-conjugated polymer hexagonal arrays, using trigonal carbon as the connecting unit, with their corresponding electronic band structures, ( a ) polyacetylene (PA)-based-C-A 3 , ( b ) polypyrene (PPyr)-based 2D-C-Pyr 3 , ( c ) polypyrrole (PPy)-based 2D-C-(Py 2 ) 3 , ( d ) Poly(p-phenylene) (PPP)-based 2D-C-(PP 2 ) 3 . The singly occupied p z state on each of the two identical carbon atoms in the unit cell act to create linear crossing bands at the Fermi level, creating a Dirac cone as for graphene. Note the oligomers are nonplanar (dihedral angles of 2D-C-A 3 =12°, 2D-C-Pyr 3 =30°, 2D-C-(Py 2 ) 3 =18°, 2D-C-(PP 2 ) 3 =30°, 2D-C-Th 3 =21°). 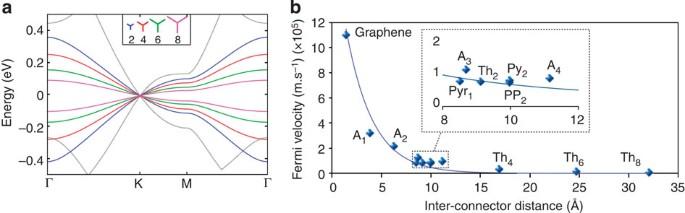Figure 4: Controlling the Fermi velocity. The oligomer chain length between carbon atom connectors controls the connector spacing and corresponding Fermi velocity of the system. (a) Electronic band dispersion around the Fermi level for single carbon atom connectors, interlinked with thiophene chains of varying length, inset key shows number of thiophene groups per chain (graphene shown for comparison in grey). (b) Fermi velocity in these 2D conjugated polymers follows an approximately inverse exponential relation to the connector spacing, largely independent of choice of interconnecting oligomer (inset shows some variations, indicative of weak electronic coupling between connectors and oligomers). Data labels refer to the interconnecting oligomer chains (seeFig. 3), exponential fity=19.59 × exp(−0.375 ×x) included as a guide for the eye. Full size image Controlling the Fermi velocity Figure 4 shows the effect of oligomer choice on the resultant 2D-CP Fermi velocity. 2D-CPs have lower Fermi velocities than that of graphene which, critically, can be precisely tuned over a wide range through appropriate oligomer choice. As such 2D-CPs should be of great interest for room temperature studies of anomalous integer Quantum Hall effect and other quantum electrodynamics phenomena [2] , [25] . At the same time these Fermi velocities remain comparable to those of conventional doped 1D-conjugated polymers such as Polymeric Tetrathiafulvalenes (PTTF) [26] , [27] . They have the additional advantages of ballistic carriers and an extended 2D network rather than hopping between finite 1D chains. This makes them highly competitive for organic electronics. The band structures of 2D-CPs also provide a potential advantage for organic electronics over graphene. The continuity of bands at the Fermi level in graphene poses problems for switching devices such as transistors, as it precludes a current ‘off’-state and requires approaches to open a band gap to render the material semiconducting. In contrast, the band structures of 2D-CPs shown here consist of crossed bands at the centre of what is otherwise a wide band gap material. This could allow for an alternative switching configuration whereby the Fermi level is displaced from the region of linear dispersion into the gap above or below these central bands. Mechanisms for Fermi level displacement are discussed further below. Figure 4: Controlling the Fermi velocity. The oligomer chain length between carbon atom connectors controls the connector spacing and corresponding Fermi velocity of the system. ( a ) Electronic band dispersion around the Fermi level for single carbon atom connectors, interlinked with thiophene chains of varying length, inset key shows number of thiophene groups per chain (graphene shown for comparison in grey). ( b ) Fermi velocity in these 2D conjugated polymers follows an approximately inverse exponential relation to the connector spacing, largely independent of choice of interconnecting oligomer (inset shows some variations, indicative of weak electronic coupling between connectors and oligomers). Data labels refer to the interconnecting oligomer chains (see Fig. 3 ), exponential fit y =19.59 × exp(−0.375 × x ) included as a guide for the eye. Full size image In a simple tight binding description, the Fermi velocity in a hexagonal array of p z orbitals is given by , where t is the nearest-neighbour effective hopping parameter and a is the lattice constant [4] . If a connector network of trigonal carbons in 2D-CPs was entirely decoupled from the oligomer states, the drop-off in hopping parameter should scale with increasing connector spacing following the form t ( a )= t 0 exp( α (( a / a 0 )−1)) (refs 28 , 29 ), where t 0 and a 0 come from pristine graphene. While we indeed find a general link between Fermi velocity and connector spacing, this appears to follow better an inverse exponential ( υ F =19.594 exp(−0.375 a ), Fig. 4 ), suggesting a more complex relationship involving the coupling of individual hopping parameters along the oligomer chains. The small deviations from the fit further reflect the coupling between the oligomer and connector networks (see Fig. 4b inset). As the oligomer chain lengths increase, the Fermi level states become increasingly localized on the connectors, with the logical limit a network of isolated quantum dots separated by long chains of semiconducting conjugated polymer. Stability and synthesis Resonance stabilization within the structure serves to chemically stabilize the trivalent carbon connectors. Our calculated binding energy for 1/2 H 2 to a triphenylmethyl monomer is 1.38 eV. However, this more than halves, to only 0.59 eV, when binding to an equivalent trivalent carbon atom in a large 993 atom supercell of 2D-C-(Ph 2 ) 3 . This result strongly suggests chemical stability in such networks. The triphenylmethyl monomer radical is already a stable persistant organic radical (at 2% concentration in benzene), which is further resonance-stabilized as shown above in the 2D-CP network. We note that these calculations also suggest a potential synthesis route, by initially stabilizing the monomeric carbon connector through functionalization and later removing the functional group once the monomers are polymerized. The binding energy of 1/2 Br 2 to triphenylmethyl, to give commercially available bromotriphenylmethane, is 1.27 eV; this drops to 0.52 eV within the extended 2D-C-(Ph 2 ) 3 layer. For a methyl group the effect is even more marked; the binding energy of 1/2 C 2 H 6 drops from 0.92 eV to the triphenylmethyl monomer, to only 0.13 eV to the 2D-C-(Ph 2 ) 3 layer. Synthesis of such materials could also be attempted through self-polycondensation of monomers such as Tris(4-bromophenyl)methanol and Tris(4-bromophenyl)phosphine. Related materials such as COP-2 have been successfully synthesized from tris(4-bromophenyl)amine monomers giving partially ordered 3D networks this way [30] , [31] . We note that geometric planarity is not a precondition to obtain such ‘Dirac-cone’ band structures. Many of the structures shown in Fig. 3 exhibit significant torsion along the polymer chains, because of steric hindrance between monomers or around the junctions (dihedral angles of 2D-C-A 3 =12°, 2D-C-Pyr 3 =30°, 2D-C-(Py 2 ) 3 =18°, 2D-C-(PP 2 ) 3 =30° and 2D-C-(Th 2 ) 3 =21°). The structures represent stable minima, for example, NPT molecular dynamics (MD) simulations find that a free-standing single layer of 2D-C-(Th 2 ) 3 retains its structure up to 700 K (at which point the chains break), showing similar high thermal stabilities to COFs [8] . In addition Fig. 5 demonstrates that the linear band crossing is conserved in the presence of a substrate (graphene in this case). Together, these results serve to demonstrate the robustness of the 2D-CP intrinsic properties for practical application. 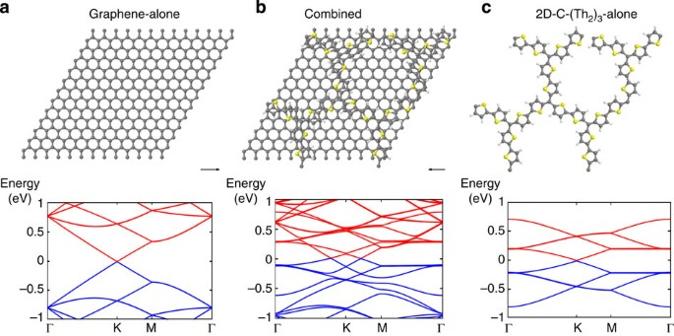Figure 5: 2D-C-Th2on a graphene substrate. (b) The 2D-conjugated polymer 2D-C-(Th2)3placed on a graphene surface and relaxed, sits an average of 3.53 Å above the graphene and shows that the linear bands are preserved at theK-point of the Brillouin zone. It can be seen that the band structure is essentially a superposition of the two independent band structures for (a) graphene and (c) 2D-C-(Th2)3. The atom colour scheme is carbon (grey), sulphur (yellow), hydrogen (white). Figure 5: 2D-C-Th 2 on a graphene substrate. ( b ) The 2D-conjugated polymer 2D-C-(Th 2 ) 3 placed on a graphene surface and relaxed, sits an average of 3.53 Å above the graphene and shows that the linear bands are preserved at the K -point of the Brillouin zone. It can be seen that the band structure is essentially a superposition of the two independent band structures for ( a ) graphene and ( c ) 2D-C-(Th 2 ) 3 . The atom colour scheme is carbon (grey), sulphur (yellow), hydrogen (white). Full size image 2D and 3D Dirac cone engineering Thus far, we have demonstrated how it is possible to create 2D arrays of conjugated polymers that mimic the electronic properties of graphene. However, the structural flexibility of these new materials gives them additional advantages beyond that of graphene. The key among these is the ability to maintain linear band dispersion when stacked into 3D layered crystals. The most stable stacking arrangement for layers of 2D-C-(Th 2 ) 3 is AA stacking with trigonal C atoms superposed at a distance of 3.14 Å (AB stacking is suppressed because of the torsion in the thiophene chains). In this case, weak interlayer coupling removes the Dirac cone, analogous to the behaviour seen in graphene/graphite ( Fig. 6 ). However, chemically modifying the polymer chains, for example, butylating the thiophene moities, sterically hinders close-packed stacking. In this case, while the system maintains AA stacking, the interlayer C–C distance at the junctions increases to 4.63 Å and the layers decouple, restoring the Dirac cone ( Fig. 6 ). This exciting possibility removes the technologically constraining requirement for isolation of individual monolayers as a prerequisite for Dirac cones, opening the way to bulk solution chemistry synthesis of 3D-layered ‘Dirac crystals’. 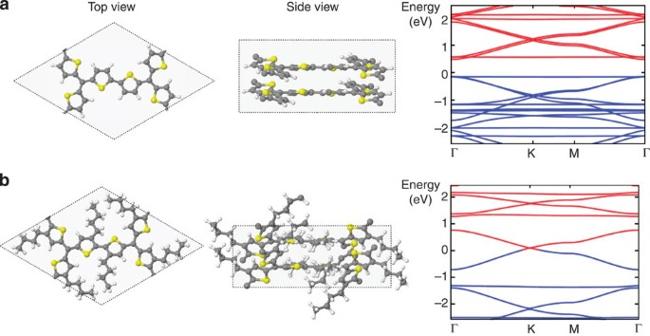Figure 6: Multilayer 2D-CPs maintaining their Dirac cone. (a) AA-stacked multilayer 2D-C-(Th2)3; the calculated interlayer spacing is 3.15 Å leading to strong interaction between layers. The respective band structure gives a small gap semiconductor material (b) AA-stacked multilayer 2D-C-(Th2)3with one hydrogen on each thiophene monomer substituted with 1-butyl group. The steric hindrance between the 1-butyl group becomes more important than the interlayer interaction and the layers are further separated from each other, decoupling the interlayer interaction between the linking carbon connectors, and restoring the Dirac cone. Figure 6: Multilayer 2D-CPs maintaining their Dirac cone. ( a ) AA-stacked multilayer 2D-C-(Th 2 ) 3 ; the calculated interlayer spacing is 3.15 Å leading to strong interaction between layers. The respective band structure gives a small gap semiconductor material ( b ) AA-stacked multilayer 2D-C-(Th 2 ) 3 with one hydrogen on each thiophene monomer substituted with 1-butyl group. The steric hindrance between the 1-butyl group becomes more important than the interlayer interaction and the layers are further separated from each other, decoupling the interlayer interaction between the linking carbon connectors, and restoring the Dirac cone. Full size image Appropriate choice of structural monomer allows an unprecedented level of band structure design, producing distorted Dirac cones with correspondingly anisotropic charge carrier Fermi velocities. Critically, this is achieved without the need for external stimuli such as electric fields [32] or applied strain [33] , [34] . By varying the length and composition of the polymer chains in the unit cell, it is possible to design lower symmetry band structures and shift and/or even merge the cones ( Fig. 7 ). Breaking the cell symmetry changes the nearest-neighbour hopping matrix elements, distorting the cones and moving them away from the K-points in the Brillouin zone. In Fig. 7c the two polyacetylene backbones have aligned, merging the cones to give a 1D metallic non-Peierls distorted conjugated polymer band structure in the k x direction, while the PTh crosslinkers maintain a residual cone structure along k y ( Supplementary Fig. 2 ). Extending the PTh lengths would complete the transition to a classical non-Peierls distorted polyacetylene band structure. 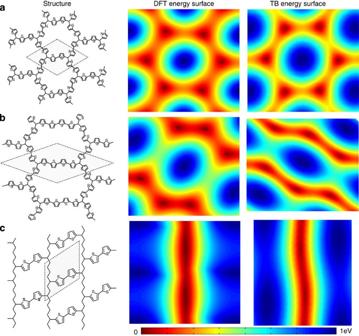Figure 7: Distorting the Dirac cones. By varying the interlinking conjugated chains, the hexagonal symmetry of the system is broken, but linear dispersion around the Fermi level is maintained. Left column shows three structures with asymmetric conjugated linkers, in each case with trigonal carbon connectors, connected via (a) 2 × Th2+Py2, (b) 2 × Th2+Th4and (c) A2+A4+Th2. Centre column shows the energy surface ink-space of the first unoccupied state from DFT-LDA calculations. In all cases a small gap is opened (A:8.0, B:7.0, C:1.0 meV). Right column shows the equivalent nearest-neighbour tight-binding (TB) energy surfaces for a hexagonal system where cell dimensions are maintained and just the effective hopping parametersγ1–3between trivalent carbon atoms are varied (A:γ1=γ2=1.1γ3, B:γ1=γ2=2.0γ3, C:γ1=γ2=8.0(γ3). These demonstrate that the energy surface behaviour is dominated by changes in the coupling between the connecting carbon atoms rather than the chain structures themselves. 3D cones are shown inSupplementary Fig. 2. The colour scale varies from dark red at the Fermi level to dark blue at +1 eV. Figure 7: Distorting the Dirac cones. By varying the interlinking conjugated chains, the hexagonal symmetry of the system is broken, but linear dispersion around the Fermi level is maintained. Left column shows three structures with asymmetric conjugated linkers, in each case with trigonal carbon connectors, connected via ( a ) 2 × Th 2 +Py 2 , ( b ) 2 × Th 2 +Th 4 and ( c ) A 2 +A 4 +Th 2 . Centre column shows the energy surface in k -space of the first unoccupied state from DFT-LDA calculations. In all cases a small gap is opened (A:8.0, B:7.0, C:1.0 meV). Right column shows the equivalent nearest-neighbour tight-binding (TB) energy surfaces for a hexagonal system where cell dimensions are maintained and just the effective hopping parameters γ 1–3 between trivalent carbon atoms are varied (A: γ 1= γ 2 =1.1 γ 3 , B: γ 1 = γ 2 =2.0 γ 3 , C: γ 1 = γ 2 =8.0( γ 3 ). These demonstrate that the energy surface behaviour is dominated by changes in the coupling between the connecting carbon atoms rather than the chain structures themselves. 3D cones are shown in Supplementary Fig. 2 . The colour scale varies from dark red at the Fermi level to dark blue at +1 eV. Full size image This can again be understood via a simple nearest-neighbour tight binding model. Varying the effective direct renormalized hopping parameters between carbon atom connectors in a hexagonal cell, following the model of [4] , [35] , we can see the three examples in Fig. 7 that represent a continuous transition between the sixfold symmetric Brillouin zone of graphene to a 1D linear band structure equivalent to metallic non-Peierls distorted polyacetylene. Heteroatoms and functionalization Other conducting connectors besides single carbon atoms, such as nitrogen and boron, demonstrate similar electronic behaviour (see Fig. 8 ). While the Dirac cone band structure is maintained, the additional nitrogen electrons raise the Fermi level well above the conical bands into the gap region above, rendering the material a wide-gap semiconductor. A partially ordered variant of this material has been successfully synthesized through self-polycondensation of tris(4-bromophenyl)amine monomers (COP-2 (refs 30 , 31 ), or 2D-N-(PP 2 ) 3 in our current notation), and indeed shows an optical gap of 2.59 eV. Approaches to lower the Fermi level to access the Dirac cones are discussed below. Metal atoms could also be used as connectors, and indeed an organometallic lattice using metal connectors has recently been proposed demonstrating Dirac cones (2D-M-(PP) 3 in our current notation, where M is a metal atom such as Pb, Bi [36] , In [37] and Mn [38] ). The increased spin–orbit coupling in these cases will result in a larger band gap. We note that a related organometallic material, Ni 3 C 12 S 12 , has been synthesized [39] and shown to produce Dirac cones [40] . In this case, however, the metal atoms serve as short linkers rather than connectors, which consist of C 6 S 6 units. As well as single-atom connectors discussed thus far, extended conjugation can also be achieved through larger ligand connectors ( Fig. 8 ). This can also be demonstrated with many different conjugated polymers, and even with noncarbon conjugated connectors such as in carbazidyl sesquisulphide (CN 2 S) [41] ( Fig. 8 ). 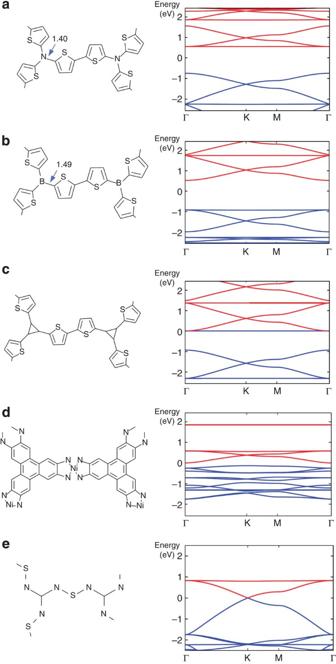Figure 8: Extending the family of 2D-CPs. Structures and band structures for (a) 2D-N-(PP2)3and (b) 2D-B-(PP2)3, the equivalent of the 2D-conjugated polymer 2D-C-(PP2)3with carbon connector atoms substituted by nitrogen and boron, respectively. The Fermi level shifts into the band gap above or below the linear dispersed bands, respectively, resulting in a wide-gap semiconductor material. (c) 2D-C3-(Tp2)3, another Dirac cone 2D-CP, uses C3structural units as connectors (d) [Ni3(2,3,6,7,10,11-hexaiminotriphenylene)2] from ref.69, whose associated band structure shows Dirac cones just below the Fermi level. (e) Carbazidyl sesquisulphide (CN2S2) proposed by Whangboet al.41, whose band structure shows a Dirac cone at the Fermi level. Bond lengths in Angstroms. Figure 8: Extending the family of 2D-CPs. Structures and band structures for ( a ) 2D-N-(PP 2 ) 3 and ( b ) 2D-B-(PP 2 ) 3 , the equivalent of the 2D-conjugated polymer 2D-C-(PP 2 ) 3 with carbon connector atoms substituted by nitrogen and boron, respectively. The Fermi level shifts into the band gap above or below the linear dispersed bands, respectively, resulting in a wide-gap semiconductor material. ( c ) 2D-C 3 -(Tp 2 ) 3 , another Dirac cone 2D-CP, uses C 3 structural units as connectors ( d ) [Ni 3 (2,3,6,7,10,11-hexaiminotriphenylene) 2 ] from ref. 69 , whose associated band structure shows Dirac cones just below the Fermi level. ( e ) Carbazidyl sesquisulphide (CN 2 S 2 ) proposed by Whangbo et al . [41] , whose band structure shows a Dirac cone at the Fermi level. Bond lengths in Angstroms. Full size image The amazing versatility of conjugated polymer chemistry can now be applied to these materials in order to tune their properties in ways not available to graphene. As for conjugated polymers, there are a number of ways to displace the Fermi level, for example, by mixing with acceptors such as I 3 ( Fig. 9b ), adding acceptor R-groups such as carboxylates to the polymer chains ( Fig. 9c ), electrochemically, or by gating the material. These drop the Fermi level of 2D-N-(PP 2 ) 3 , converting the material from wide-gap semiconductor, through conventional metallic conductor, to a ballistic conductor in the linear regime. In addition, carboxylate functionalization renders the Fermi level of the network pH-dependent. Such switchable materials could serve as transistors, controlling the Fermi level via an external gate, or as highly sensitive electrochemical detectors. Copolymer linking chains could be used, and functionalization with porphyrins and other side groups could also be used to add dynamic response to the network such as optical switching, light harvesting or emission and gas detection. This direct link between chemical design and dynamic electronic response makes these materials highly attractive as carbon-based electronic platforms [42] . Their low mass and optical density suggest further applications such as transparent conductive membranes. 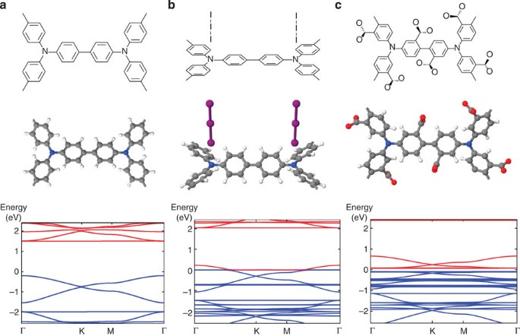Figure 9: Tuning the Fermi level of 2D-conjugated polymers. (a) 2D-N-(PP2)3, the equivalent of the 2D-conjugated polymer 2D-C-(PP2)3with carbon connector atoms substituted by nitrogen. The additional nitrogen electrons shift the Fermi level into the band gap above the linear dispersed bands, resulting in a wide-gap semiconductor material. 2D-CPs can be doped in various ways, such as (b) the presence of I3extracts electrons and renders 2D-N-(PP2)3metallic, (c) carboxylate functionalization of the phenylene rings allows for pH-dependent displacement of the Fermi level, in this case displaced below the nitrogen atom Dirac cone states. Only the unit cells are shown here. Figure B is tilted compared with A and B for better perspective. Iodine atoms are in purple and oxygen atoms in red. Figure 9: Tuning the Fermi level of 2D-conjugated polymers. ( a ) 2D-N-(PP 2 ) 3 , the equivalent of the 2D-conjugated polymer 2D-C-(PP 2 ) 3 with carbon connector atoms substituted by nitrogen. The additional nitrogen electrons shift the Fermi level into the band gap above the linear dispersed bands, resulting in a wide-gap semiconductor material. 2D-CPs can be doped in various ways, such as ( b ) the presence of I 3 extracts electrons and renders 2D-N-(PP 2 ) 3 metallic, ( c ) carboxylate functionalization of the phenylene rings allows for pH-dependent displacement of the Fermi level, in this case displaced below the nitrogen atom Dirac cone states. Only the unit cells are shown here. Figure B is tilted compared with A and B for better perspective. Iodine atoms are in purple and oxygen atoms in red. Full size image A related family of previously proposed monolayer materials are graphynes [43] , [44] and graphdiynes [43] . While these are likely to be chemically reactive, predictions of Dirac cones in graphyne and graphdyene phases [5] , [35] should be structurally transferable to 2D-CPs. Other diverse ‘graphene variants’ featuring square and decagonal motifs [45] , while unstable in pure carbon, will have 2D-CP analogues. Notable among 2D-Euclidean tilings are Kagome acute lattices [46] with a combination of linear dispersion and structurally localized states [47] , which could be produced this way. This diversity of structural motifs further increases the range of potential 2D-conjugated polymeric structures with massless Dirac fermions. This paper demonstrates a new family of 2D networks of conjugated polymers with linear band dispersion at or near the Fermi level. These should be possible to synthesize utilizing synthesis strategies developed for COFs and related organic frameworks, indeed already demonstrated experimentally for 2D-N-(PP 2 ) 3 . Their physical and electronic structure remains robust to high temperatures, both free-standing, on substrates, and in layered crystals. Given the range of potential 2D architectures, chemical constituents and functional modifications, 2D-CP networks should be highly flexible and adaptable to a wide range of fundamental and applied problems. Electronic Structure Calculations Density functional (DFT) calculations were performed with the AIMPRO code, using local density (LDA-PW92) (ref. 51 ) and generalised gradient (GGA-PBE) exchange-correlation functionals and the VASP code using hybrid HSE06 (refs 55 , 56 ) functionals. For the AIMPRO calculations, relativistic pseudopotentials are generated using the Hartwingster–Goedecker–Hutter scheme [57] . Charge density was fitted with plane waves with energy cutoff 150 Ha. Electronic levels were filled using a Fermi occupation function with kT =0.01 eV. Periodic boundaries were applied with interlayer vacuum distance >10 Å for single layers. For multilayers, interlayer spacing was reduced to 3.10 Å before lattice optimization. A fine k -point grid of at least 8 × 8 × 1 for monolayer, and at least 5 × 5 × 2 for multilayer, were chosen using the Monkhorst–Pack scheme [58] . Energies are converged to better than 10 −7 Ha. Atomic positions and lattice parameters were geometrically optimized before band structure calculations with basis sets of 38/12/40 independent Gaussian functions for carbon/hydrogen/other heteroatoms. VASP calculations, with electron–core interactions represented by the projector-augmented wave approximation [59] , [60] . The plane-wave cutoff was 400 eV, with Methfessel–Paxton partial occupancies for each wavefunction. Energies are converged to better than 10 −5 Ha. Full HSE06 lattice and geometries optimization were performed before band structure calculations. The tight binding calculations were performed using PythTB ( http://www.physics.rutgers.edu/pythtb/index.html ). Molecular dynamics The classical MD code was LAMMPS [61] , [62] , with the ReaxFF potential [63] . The runs were carried out for 6 ns with time step of 0.1 fs. Time integration (10 fs) was used on Nose–Hoover [64] , [65] style non-Hamiltonian equations of motion, designed to generate positions and velocities sampled from the canonical (nvt) method (constant volume and temperature), using the same supercells as for the DFT calculations. Test models of 1D-PTh found chain breakdown between 900 and 1,000 K, matching experimental thermogravimetric analysis (TGA) measurements of 973±100 K (ref. 66 ). How to cite this article: Adjizian, J.-J. et al . Dirac Cones in two-dimensional conjugated polymer networks. Nat. Commun. 5:5842 doi: 10.1038/ncomms6842 (2014).